Adaptive strong-field control of chemical dynamics guided by three-dimensional momentum imaging Shaping ultrafast laser pulses using adaptive feedback can manipulate dynamics in molecular systems, but extracting information from the optimized pulse remains difficult. Experimental time constraints often limit feedback to a single observable, complicating efforts to decipher the underlying mechanisms and parameterize the search process. Here we show, using two strong-field examples, that by rapidly inverting velocity map images of ions to recover the three-dimensional photofragment momentum distribution and incorporating that feedback into the control loop, the specificity of the control objective is markedly increased. First, the complex angular distribution of fragment ions from the nω +C 2 D 4 →C 2 D 3 + +D interaction is manipulated. Second, isomerization of acetylene ( nω +C 2 H 2 →C 2 H 2 2+ →CH 2 + +C + ) is controlled via a barrier-suppression mechanism, a result that is validated by model calculations. Collectively, these experiments comprise a significant advance towards the fundamental goal of actively guiding population to a specified quantum state of a molecule. Chemical reaction dynamics can be monitored on timescales of the electronic and nuclear motions [1] , [2] , [3] , [4] , [5] , [6] , [7] , thanks to advances in laser technology [7] , [8] , [9] . These advances have led to increasing interest in using ultrafast laser pulses to manipulate chemical processes via direct control of the electronic and nuclear dynamics [7] , [10] . Active manipulation of the dynamics, however, is a challenging problem: rapid internal vibrational redistribution often thwarts simple approaches; the laser-modified potential energy surfaces (PESs) are complex; and the intense laser-molecule interaction must not destroy the target system before it reaches its desired final state. For these reasons and others, a priori selection of suitable laser-pulse characteristics remains an intractable problem for all but the simplest reactions. Adaptive femtosecond control has proved to be a powerful alternative strategy [11] , [12] , [13] , [14] . In adaptive femtosecond control, a learning algorithm uses experimental feedback to change the parameters defining the laser pulse shape and thereby iteratively approaches the desired control objective, effectively solving the Schrödinger equation in real time [12] . This approach circumvents the need for detailed knowledge of the nonlinear response of the molecule to the laser field, but the complexity of the resulting optimal pulses often obscures the mechanism driving the control. Disentangling the pulse complexities to arrive at mechanistic insight remains relatively rare (for example refs 14 , 15 , 16 ), especially in the strong-field regime and in experiments that lack precise spectroscopic feedback signals. Improving the understanding of the control mechanism provides fundamental information about the complex laser-molecule dynamics, thus revealing behaviour that will build the physical intuition necessary to properly parameterize the large multi-dimensional phase space defining the pulse shape [17] , [18] . The learning algorithm often needs several thousand trial pulses to converge on a solution, and therefore often a simple product yield (for example, time-of-flight mass spectrometry) is employed to obtain rapid feedback. Although these signals can be obtained quickly, the control target is often ambiguous. Moreover, most successful examples of reverse engineering the pulse characteristics involve the interplay between careful parameterization of the search space and detailed spectroscopic feedback [14] , [15] , [19] , whereas similar attempts using ion yields have been less successful [18] . Various multi-dimensional ion imaging techniques can provide spectroscopic level discernment [20] , [21] , but they have been too slow for adaptive control and have not been implemented so far. In this Article, we demonstrate the use of a rapid three-dimensional (3D) momentum imaging technique that is incorporated directly into the feedback loop for adaptive control of molecular dynamics. Two primary examples are presented. In the first, image-based feedback allows manipulation of the angular distributions of photofragments arising from strong-field ionization of ethylene, a non-linear molecule with a rich spatial pattern. This example demonstrates the ability of 3D image-based feedback to target and control objectives that are not typically accessible using standard time-of-flight or spectroscopic techniques. In the second example, we control the isomerization dynamics in the doubly charged ions of acetylene. Beyond the control itself, the 3D image-based feedback has stimulated theoretical calculations that identify the barrier-suppression mechanism responsible for increasing the isomerization yield. Furthermore, this control solution has proved robust, with different searches reaching essentially similar pulse characteristics despite different pulse parameterization schemes. On the basis of this range of initial results, we surmise that the use of multi-dimensional momentum feedback opens new avenues for exploration using adaptive control, especially in complex systems or when spectroscopic feedback is impractical. Experiment As detailed in the Methods section, the image-based feedback was obtained by employing velocity map imaging (VMI) [22] in combination with a rapid inversion algorithm for online 3D feedback. Although past work has combined strong field pulse shaping with imaging [23] , [24] , [25] , and a few previous efforts [26] , [27] , [28] , [29] used VMI for adaptive control, they were exclusively based on raw images, in which the 3D momentum distributions were projected onto the two-dimensional (2D) detector plane. The azimuthal ambiguity inherent in such raw, 2D images complicated the extraction of a robust feedback signal [26] . Previous inversion methods to obtain slices through the 3D momentum distribution were often too slow to be practical for adaptive control or depended critically on selecting initial parameters (such as the correct basis set for transformation) before the inversion. By implementing a rapid onion-peeling algorithm [30] , the inversion time for a 1,050 × 1,024 pixel image was reduced to less than one second, thus enabling 3D momentum feedback for adaptive control. Ethylene Our first control example applies 3D image-based feedback to strong-field ionization of ethylene, specifically the complex angular dependence of C 2 D 3 + ions produced by deuterium atom elimination ( nω +C 2 D 4 →C 2 D 3 + +D). This process produces the inner four-lobed structure, shown in Fig. 1a , whereas the outer ring structure has a momentum that matches a similar structure on the D + VMI data, suggesting that it is associated with the double ionization channel ( nω +C 2 D 4 →C 2 D 3 + +D + ). As the lobes associated with C 2 D 3 + +D are neither perpendicular nor parallel to the polarization direction, extracting this weak channel from time-of-flight mass spectrometry would be difficult. Even the use of raw, 2D VMI is problematic, as azimuthal contributions from the dominant outer double-ionization ring would obscure the inner structure. The 3D momentum feedback allows extraction of the angle-resolved yield from the regions shown in Fig. 1a , which subsequently define the control objective. 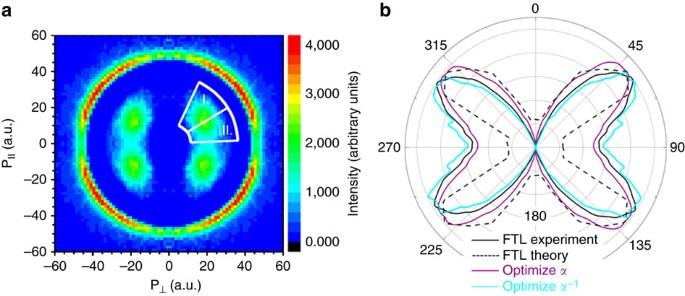Figure 1: C2D3+photofragment image and angular distribution. (a) Measured momentum distribution (in atomic units) of C2D3+fragments following ionization by near FTL 45 fs duration laser pulses centred at 782 nm with a peak intensity of 2 × 1015W cm−2. The laser polarization direction is vertical in all panels. The more intense outer structure has a similar shape and momentum to that observed in the D+VMI data, and is therefore assumed to be associated with the C2D3++D+channel. The inner structure has no similar momentum matching partner, and is thus associated with C2D4+→C2D3++D. The white lines define the two regions from which yields were extracted to determineα, the control objective. (b) A comparison of the measured angular distributions for strong-field ionization by different optimized pulses leading to C2D4+→C2D3++D. Violet represents the distribution obtained by maximizingαand cyan arises from maximizingα−1. In these experiments,αincreased by 65% over the value with a FTL pulse. To put this number in context, we note that over the duration of the search process, the fitness value obtained with FTL pulses fluctuated with a standard deviation (σ) of 5% around the average value, and thus the enhancement ofσrelative to the value obtained with the near-FTL pulse level equates to 13σ.α−1was increased by 22% or 6σ. In black is the comparison between experimental (solid) and theoretical (dashed) angle-resolved ionization probabilities for the C2D4+→C2D3++D process shown inFig. 1a. Figure 1: C 2 D 3 + photofragment image and angular distribution. ( a ) Measured momentum distribution (in atomic units) of C 2 D 3 + fragments following ionization by near FTL 45 fs duration laser pulses centred at 782 nm with a peak intensity of 2 × 10 15 W cm −2 . The laser polarization direction is vertical in all panels. The more intense outer structure has a similar shape and momentum to that observed in the D + VMI data, and is therefore assumed to be associated with the C 2 D 3 + +D + channel. The inner structure has no similar momentum matching partner, and is thus associated with C 2 D 4 + →C 2 D 3 + +D. The white lines define the two regions from which yields were extracted to determine α , the control objective. ( b ) A comparison of the measured angular distributions for strong-field ionization by different optimized pulses leading to C 2 D 4 + →C 2 D 3 + +D. Violet represents the distribution obtained by maximizing α and cyan arises from maximizing α −1 . In these experiments, α increased by 65% over the value with a FTL pulse. To put this number in context, we note that over the duration of the search process, the fitness value obtained with FTL pulses fluctuated with a standard deviation ( σ ) of 5% around the average value, and thus the enhancement of σ relative to the value obtained with the near-FTL pulse level equates to 13 σ . α −1 was increased by 22% or 6 σ . In black is the comparison between experimental (solid) and theoretical (dashed) angle-resolved ionization probabilities for the C 2 D 4 + →C 2 D 3 + +D process shown in Fig. 1a . Full size image The control objective, α ≡ N I / N II , was defined in terms of a ratio of the yields ( N ) in the two regions (labelled I and II) shown in Fig. 1a . Optimizing α , or selecting laser pulse shapes to shift the angular distributions towards the polarization direction, led to a 65% enhancement of the control objective. This increase was 13 times greater than the level of random fluctuations in the experiment ( σ ). The resulting angular distribution is shown in Fig. 1b . Moving the angular distribution away from the polarization angle (that is, optimizing α −1 ) as shown in Fig. 1b , proved harder, with an enhancement of 22% (6 σ ). Acetylene The second example of the 3D image-based control technique involves strong-field isomerization of acetylene dications. Isomerization is monitored by examining the CH 2 + and CH + ion images from the laser-induced fragmentation of the molecule. Previous coincidence measurements [31] , [32] indicated that CH 2 + ions are associated with a vinylidene-like configuration of the dication, whereas CH + ions are the result of double ionization leading to a symmetric CH + +CH + breakup from the acetylene configuration. The migration of the hydrogen in the former process imparts a significant angular momentum to the molecule, producing a nearly isotropic distribution of ions [32] . The symmetric breakup of acetylene-like [HCCH] 2+ , however, occurs predominately along the laser polarization direction. The CH 2 + and CH + angular distributions obtained in our experiments are displayed in Fig. 2 , showing the probability density as a function of both the fragment kinetic energy release (KER) and cos θ , where θ is the angle between the ion momentum and the laser polarization axis. The earlier acetylene work [31] , [32] suggested that the regions shown by the white lines in Fig. 2a,b,d,e be used to define the vinylidene/acetylene ratio. 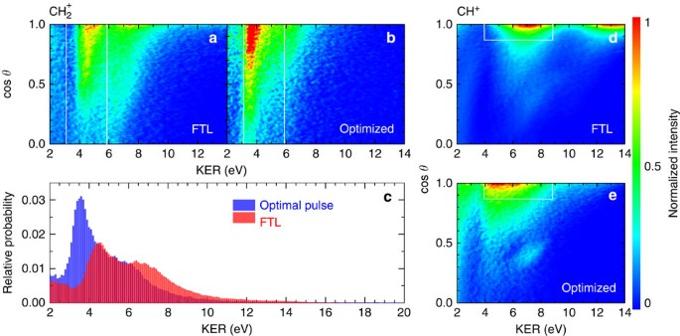Figure 2: CH2+and CH+photofragment data. Measured density plots of dissociating CH2+(aandb) and CH+(dande) ions as a function of KER and cosθfor FTL pulses (aandd) and pulses optimized to enhance the CH2+channel (bande). The white boxes in the density plots define the regions used to obtain the CH2+and CH+yields used in the control objective. As shown in (c), the probability of dissociation as a function of KER for CH2+ions reveals that laser pulses tailored to enhance the angle-resolved CH2+/CH+ratio produce CH2+ions with a KER distribution that peaks at more than 1 eV lower than the distribution obtained with FTL pulses. The FTL pulses have a centre wavelength of 778 nm, a FWHM duration of 45 fs and a focused intensity of ≈8 × 1014W cm−2. Each density plot is normalized to the peak intensity for that particular exposure and displayed with the same linear colour scale (shown at right) for each image. Figure 2: CH 2 + and CH + photofragment data. Measured density plots of dissociating CH 2 + ( a and b ) and CH + ( d and e ) ions as a function of KER and cos θ for FTL pulses ( a and d ) and pulses optimized to enhance the CH 2 + channel ( b and e ). The white boxes in the density plots define the regions used to obtain the CH 2 + and CH + yields used in the control objective. As shown in ( c ), the probability of dissociation as a function of KER for CH 2 + ions reveals that laser pulses tailored to enhance the angle-resolved CH 2 + /CH + ratio produce CH 2 + ions with a KER distribution that peaks at more than 1 eV lower than the distribution obtained with FTL pulses. The FTL pulses have a centre wavelength of 778 nm, a FWHM duration of 45 fs and a focused intensity of ≈8 × 10 14 W cm −2 . Each density plot is normalized to the peak intensity for that particular exposure and displayed with the same linear colour scale (shown at right) for each image. Full size image The KER distribution of CH 2 + ions obtained with a Fourier-transform limited (FTL) pulse is peaked at 4.85 eV, consistent with previous coincidence measurements of the C + +CH 2 + dissociative double-ionization channel, which show a sharply-peaked distribution near 5 eV that is nearly independent of cos θ (refs 31 , 32 ). The CH + fragments peaked at around 7 eV along the polarization direction are consistent with previous measurements of the C 2 H 2 2+ dissociation into CH + +CH + , whereas the higher KER features are assumed to arise from higher charge states of the parent molecule. When the learning algorithm was allowed to adjust the pulse shape, the angle-resolved target ratio of CH 2 + /CH + could be either almost doubled (40 σ ) or suppressed to half of the original value (25 σ ) over a range of laser pulse energies. Interestingly, the KER obtained with the pulse optimized to enhance the isomerization channel showed a downward shift to 3.6 eV and suppression of the high KER feature around 7 eV. As illustrated in Fig. 3 , measurement of these optimized pulses with a SHG FROG [33] showed that the individual pulse characteristics have little similarity aside from a need for multiple peaks spaced by 100–210 fs. 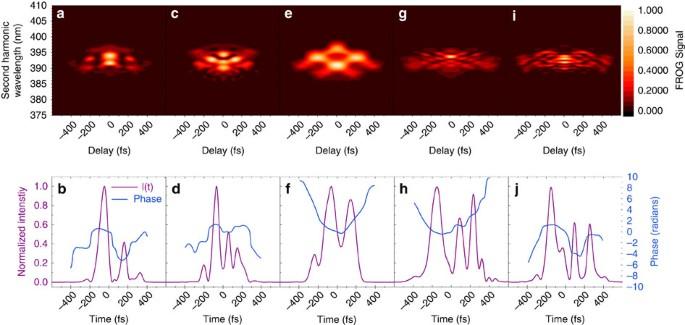Figure 3: Laser pulse characterization. SHG FROG30measurements (top) and the associated intensity and temporal phase (bottom) for different experimental trials. (a,b) Optimized pulse using phase-only frequency domain shaping at 68 μJ per pulse obtaining 55% enhancement of the CH2+/CH+ratio. (c,d) and (e,f) are similar but at 130 μJ and again at 68 μJ pulse energy, obtaining 92% and 44% enhancement, respectively. (g,h) Results from phase-only time-domain shaping at 60 μJ per pulse, obtaining 90% enhancement. The final pulse (i,j) is manually designed and achieved 40% enhancement. Figure 3: Laser pulse characterization. SHG FROG [30] measurements (top) and the associated intensity and temporal phase (bottom) for different experimental trials. ( a , b ) Optimized pulse using phase-only frequency domain shaping at 68 μJ per pulse obtaining 55% enhancement of the CH 2 + /CH + ratio. ( c , d ) and ( e , f ) are similar but at 130 μJ and again at 68 μJ pulse energy, obtaining 92% and 44% enhancement, respectively. ( g , h ) Results from phase-only time-domain shaping at 60 μJ per pulse, obtaining 90% enhancement. The final pulse ( i , j ) is manually designed and achieved 40% enhancement. Full size image The angle-resolved ethylene data, showing increased ionization when the polarization is aligned with the C–D bond, gives insight into the ionization process. In a molecular context, the angular distribution of the strong-field ionization events are often understood in terms of the molecular orbitals involved [34] , [35] , [36] , [37] , [38] , [39] . Early theoretical efforts concentrated on ionization from the HOMO [34] , but later studies showed that when occupied valence orbitals have similar energies, both the HOMO and the HOMO-1 states can contribute to the ionization [35] , [36] , [37] , [38] . As the energy gap between orbitals decreases in polyatomic molecules, more orbitals are expected to contribute. The pattern shown in Fig. 1a can be understood by extending the calculations of angle-resolved ionization rates of diatomic molecules, described in ref. 39 , to polyatomic molecules. The neutral C 2 D 4 molecules in our effusive jet source are randomly oriented, and thus the interaction between the laser field and the electronic wavefunction depends on their relative angle. When the laser polarization is either parallel or perpendicular to the C=C backbone, the HOMO, LUMO and HOMO-1 orbitals are only slightly distorted. When the laser polarization is aligned with the C–D bond direction, however, the electron density becomes much more pliable. The result is a strongly distorted Rydberg orbital located near the deuterium atom. In this configuration, the field easily shifts electron density in that direction and the ionization rate correspondingly increases. As shown in Fig. 1b , the measured and calculated angle-resolved ionization probabilities are in reasonable agreement for FTL pulses. From a control perspective, then, modification of the angular distribution of C 2 D 3 + fragments is related to the ability of the pulse to influence the location of this Rydberg orbital. Without image-based feedback, this task would be impossible. Moreover, the C 2 D 3 + images provide experimental verification of the theoretical predictions suggesting that multiple orbitals, including the distorted Rydberg orbital, have important roles in the ionization of unsaturated hydrocarbons. In a larger sense, this example is significant because it illustrates the link image-based feedback can provide between tunnelling ionization and molecular structure. The lobe structures in this example should be present at appearance intensities because the tunnelling rates are highest where the electron cloud has the largest extent [34] . Dissociation channels such as nω +C 2 D 4 →C 2 D 3 + +D that are energetically accessible at the lowest intensity are therefore the best channels for probing and learning how to control molecular structure. Extending this link to the pulse characteristics in this case is still under investigation. Enhancing α was accomplished via a pulse that had some modulation of the spectral intensity but was only slightly longer in duration than the FTL pulse. The pulse that maximized α −1 has complicated phase characteristics and a more complex structure. In the acetylene experiment, however, the image-based feedback stimulated model calculations that yielded an understanding of the mechanism driven by the optimized laser pulse. To shed light on the molecular dynamics and time scales involved, we performed semiclassical on-the-fly calculations in full dimension for the doubly charged acetylene ion. The simulation started just after the ionization event and included the ground state and the first singlet state of C 2 H 2 2+ . Interactions with both FTL and optimized laser fields were considered. The details for the full dimension trajectory calculations are given in the Methods section. To visualize the dynamics, the full dimension trajectories have been projected onto a 2D PES spanned by the most significant reaction coordinates. This reaction PES includes all critical points, such as minima and barriers along the pathway, and shows both fragmentation channels used as the defined control objective (CH 2 + /CH + ). The first coordinate corresponds to the H migration, which can be followed in the CCH angle. The second coordinate is the CC distance leading to either the CH 2 + +C + or CH + +CH + fragmentations, depending on the CCH angle. The ab initio PES calculation, as well as the on-the-fly trajectories, used high level electron correlation theory and is shown in Fig. 4 . 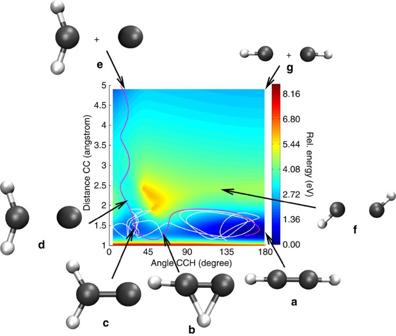Figure 4: C2H22+PES and sample trajectories. The 2D PES of the acetylene dication for the two coordinates CCH angle and CC distance. Important geometries (labelleda–g) are marked on the surface with black arrows linked to corresponding ball-and-stick structures. Point (a) on the surface represents the initial linear acetylene state, (b) represents the intermediate transition state and (c) represents the vinylidene configuration of the C2H22+dication. Dissociation from the vinylidene configuration is shown at points (d) and (e), whereas direct dissociation from the acetylene configuration proceeds through points (f) and (g). Two example trajectories are projected onto these coordinates. The white trajectory is calculated without additional laser interaction following the double ionization step and moves only between the structures (a) over (b) to (c). The violet trajectory includes the effect of the optimized laser pulse and progresses from configuration (a) over (b) to (c) and dissociates to (d) and finally (e) because the laser interaction suppresses the barrier in the region near configuration (d). Figure 4: C 2 H 2 2+ PES and sample trajectories. The 2D PES of the acetylene dication for the two coordinates CCH angle and CC distance. Important geometries (labelled a – g ) are marked on the surface with black arrows linked to corresponding ball-and-stick structures. Point ( a ) on the surface represents the initial linear acetylene state, ( b ) represents the intermediate transition state and ( c ) represents the vinylidene configuration of the C 2 H 2 2+ dication. Dissociation from the vinylidene configuration is shown at points ( d ) and ( e ), whereas direct dissociation from the acetylene configuration proceeds through points ( f ) and ( g ). Two example trajectories are projected onto these coordinates. The white trajectory is calculated without additional laser interaction following the double ionization step and moves only between the structures ( a ) over ( b ) to ( c ). The violet trajectory includes the effect of the optimized laser pulse and progresses from configuration ( a ) over ( b ) to ( c ) and dissociates to ( d ) and finally ( e ) because the laser interaction suppresses the barrier in the region near configuration ( d ). Full size image To reach CH 2 + +C + fragmentation (e), a molecule starting from the linear configuration (a) has to pass the transition state (b). It forms a vinylidene-like local minimum geometry at (c) before dissociating over a second barrier (d) to the fragments (e). The second pathway leading to the CH + -fragments includes mostly the CC-bond elongation and is reached after crossing the barrier (f). Two example trajectories for isomerization, projected onto the 2D surface, are shown in Fig. 4 for calculations with (violet line) and without (white line) the optimized laser field. The white trajectory oscillates for some time around the acetylene-like structure (a) before overcoming the barrier to the vinylidene-like geometry. These types of trajectories do not have enough energy to cross the dissociation barrier and either remain in this configuration or return to (a). The violet trajectory moves very swiftly from geometry (a) over the suppressed barrier (b) to (c) and finally dissociates to (d) without staying long at any given structure. Most of the more than 1,000 trajectories without the optimized laser interaction stayed at structure (a) or moved between (a) and (c). Between 100 and 210 fs, trajectories with geometry (c) had the highest probability. This time period matches the time separation of the sub-pulses in the optimized field, and it appears that the second sub-pulse is timed to interact when most molecules are in configuration (c). The laser interaction shifts the PES, suppressing the dissociation barrier towards the CH 2 + fragments, allowing molecules with lower kinetic energy to cross. The theoretical KER spectrum, shown in Fig. 5 , supports this explanation and shows the same shift to a lower KER distribution as observed experimentally. Furthermore, the CH + fragments also show a shift to lower KER (see Fig. 2d,e ), which can be interpreted as a lowering of the barrier between points (a) and (g) in the PES. This barrier, however, is higher than the barrier between (c) and (d), and thus dissociation from the vinylidene configuration is expected to be favored, consistent with the experimental observations. 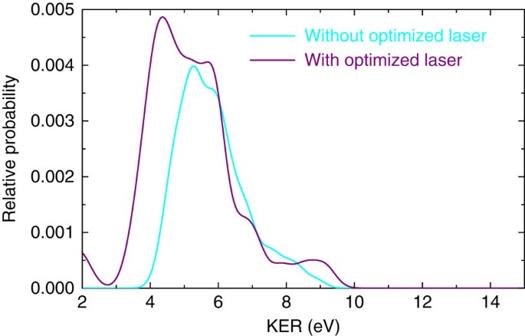Figure 5: Calculated KER spectrum for CH2+fragments. In cyan is the probability as a function of KER derived from trajectories evolving without the optimized laser pulse, that is, the calculation assumes that a near-FTL pulse accomplishes the double ionization and the subsequent wavepacket propagation is field-free. In violet is the KER spectrum associated with trajectories evolving in the presence of the optimized laser pulse that modifies the PES. In both the experiment (seeFig. 2c) and calculations, the optimized pulse opens an additional contribution at lower KER. Figure 5: Calculated KER spectrum for CH 2 + fragments. In cyan is the probability as a function of KER derived from trajectories evolving without the optimized laser pulse, that is, the calculation assumes that a near-FTL pulse accomplishes the double ionization and the subsequent wavepacket propagation is field-free. In violet is the KER spectrum associated with trajectories evolving in the presence of the optimized laser pulse that modifies the PES. In both the experiment (see Fig. 2c ) and calculations, the optimized pulse opens an additional contribution at lower KER. Full size image To further examine this isomerization mechanism, we employed phase-only shaping with a time-domain pulse parameterization [18] , rather than the standard frequency-domain parameterization used in the previously described experiments. In this scheme, our optimal pulse is built out of a series of Gaussian shaped pulses and the parameters controlled by the learning algorithm are the duration, amplitude and separation between the individual pulses. Using this parameterization and a set of three Gaussian pulses (see Fig. 3g,h ), we were again able to double the CH 2 + /CH + ratio. The reduced parameter set also converges to a solution much faster (five generations) than the original frequency domain method (≈20 generations). Importantly, the multiple-pulse solution appears general. The Dazzler pulse shaper [40] can also be used to shape the pulse manually by adjusting laser parameters such as the chirp or pulse duration. Investigations along these lines produced some minimal variation in the CH 2 + to CH + production ratio, but no simple pulse parameter could be manipulated to produce results comparable to those obtained using adaptive control. On the basis of the pulse-train features we observed in pulses optimized to enhance the isomerization ratio in acetylene, we manually designed a pulse with these important characteristics. Although it exceeded the transform-limited result, our pulse did not perform as well as the algorithm-based optimal pulse. The manually-constructed pulse train, shown in Fig. 3i,j) , produced a CH 2 + /CH + ratio 40% higher than the FTL value at 60 μJ/pulse, whereas various optimized pulses reached 90% or a greater enhancement of the ratio. Still, this result demonstrates that the 3D VMI-based feedback contains enough clues about the control dynamics to interpret the essential features of the pulse, even without using complicated numerical methods such as principal control analysis [18] , [41] , [42] . This allowed the selection of a reduced parameter set that provided as much control as the larger original basis. Gaining enough mechanistic insight to understand how to choose a useful parameter space is a key step for improving control fidelity. To verify the need for 3D momentum imaging feedback for achieving this result, we have performed the acetylene experiment using regions of the images designed to mimic a mass spectrometer with a small solid angle. In these experiments, an enhancement of the CH 2 + /CH + ratio was observed, but the result was an angular discrimination artifact, similar to what has been observed for the strong-field dissociative ionization of CO [26] . The use of the full momentum imaging as a feedback for the coherent control algorithm was thus crucial in finding the barrier-suppression mechanism. Some of the most exciting examples of adaptive control (for example refs 14 , 15 , 43 , 44 ) depend on very specific optical feedback. Collectively, the examples described above show that 3D momentum imaging feedback brings similar capabilities to ion-based experiments. The twin benefits of this approach are illustrated in our experiments: first, 3D image-based control allows the selection of well-defined control targets; second, the abundant information contained in the feedback signal can give insight into the control mechanism. In the acetylene example, the adaptive search persistently arrived at the multi-pulse barrier-suppression isomerization mechanism despite different initial parameterizations of the search space. This insensitivity to the initial parameterization indicates a high degree of control fidelity. The ethylene examples illustrate how angle-resolved feedback is crucial for the control of polyatomic systems. The general applicability of full momentum-imaging-based feedback for the adaptive control of chemical reaction dynamics promises to uncover novel control mechanisms for even more complex chemical reactions. Furthermore, strong-field processes in atoms, clusters and nanoparticles may be selectively controlled, and the resulting images may provide richly detailed information about the control mechanisms. General experimental details The core of the experiment was a closed-loop system that produces shaped, intense ultrafast laser pulses, which ionize and fragment the target molecules, producing a feedback that drives the optimization of the pulse shapes. The intensity of these pulses was sufficient to ionize either acetylene or ethylene multiple times and produce transient modifications of their PESs. The resulting photofragments were imaged with a VMI apparatus. This ion image was processed online (as described later) and a particular ‘fitness’ value was extracted, which was used by the learning algorithm to produce a new set of pulse shapes for testing. The Dazzler pulse shaper may be operated in modes that shape either the spectral phase or amplitude independently or together. In these experiments, we only shaped the phase, and thus the pulse energies remained approximately constant over the duration of an experiment. The system was linked by a computer control that connected the AOPDF pulse shaper, the learning algorithm, the digital delay generator that triggered the high-voltage switch for the microchannel plates (MCPs) and the camera readout electronics. This is illustrated schematically in Fig. 6 . 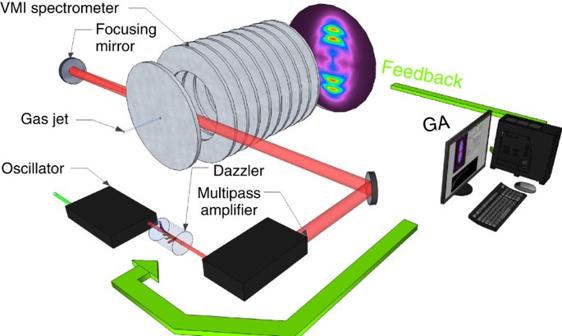Figure 6: Schematic diagram of the apparatus and the control loop. Laser pulses centered at approximately 780 nm were produced with a Ti:sapphire oscillator, shaped with an acousto-optical programmable dispersive filter37and then amplified to energies typically between 0.01 and 0.5 mJ per pulse by a multipass amplifier running at 2 kHz. The near-FTL pulses had durations of approximately 40–45 fs and, after they were focused by a (f=75 mm) spherical mirror, achieved peak intensities of approximately 2 × 1016W cm−2. The pulses intersected an effusive jet of target gas, similar to the one described in ref.42. The spectrometer electric fields were configured so that trajectories corresponding to a particular initial velocity arrived at the same position on the detector plane, even if the ions had been created at different locations within the laser focus43. The ions struck the detector MCP stack, producing an electron shower on a phosphor screen that was imaged by a CCD camera. The MCP assembly was fully powered only at times corresponding to the arrival of a single preselected ion species using a triggered high-voltage switch. The image was processed and the feedback delivered to the learning algorithm, which created the next set of pulse shapes to test. Figure 6: Schematic diagram of the apparatus and the control loop. Laser pulses centered at approximately 780 nm were produced with a Ti:sapphire oscillator, shaped with an acousto-optical programmable dispersive filter [37] and then amplified to energies typically between 0.01 and 0.5 mJ per pulse by a multipass amplifier running at 2 kHz. The near-FTL pulses had durations of approximately 40–45 fs and, after they were focused by a ( f =75 mm) spherical mirror, achieved peak intensities of approximately 2 × 10 16 W cm −2 . The pulses intersected an effusive jet of target gas, similar to the one described in ref. 42 . The spectrometer electric fields were configured so that trajectories corresponding to a particular initial velocity arrived at the same position on the detector plane, even if the ions had been created at different locations within the laser focus [43] . The ions struck the detector MCP stack, producing an electron shower on a phosphor screen that was imaged by a CCD camera. The MCP assembly was fully powered only at times corresponding to the arrival of a single preselected ion species using a triggered high-voltage switch. The image was processed and the feedback delivered to the learning algorithm, which created the next set of pulse shapes to test. Full size image Rapid inversion In this control scheme, accurate feedback from the velocity map image, in the form of an ion yield from a particular portion of the image, often depends critically on the conversion of the 2D raw image to a slice through the centre of the full 3D momentum distribution. An example is displayed in Fig. 7 , which shows the raw and inverted images of CD 3 + ions produced in a laser-ethylene interaction. Although the outer structure is visible in the raw image on the left, the inner structure is nearly completely obscured by an unwanted azimuthal contribution that can easily lead to sub-optimal control results [26] . 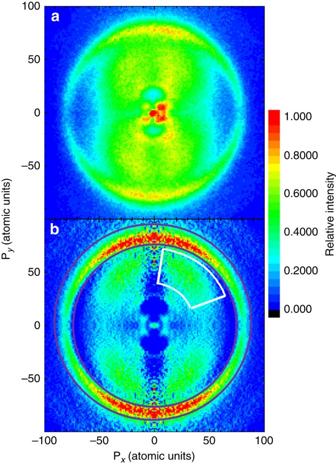Figure 7: Comparison of raw 2D and processed 3D images. The raw (a) and rapidly inverted (b) images for CD3+ions. The inversion was accomplished with the ‘onion-peeling’ or ‘back-projection’ method described in this section. The purple and white boxed regions in (b) illustrate how different processes could be isolated from the CD3+images and the corresponding yields used to define a control objective. On a 661 × 661 pixel test image, our algorithm could produce an inverted image in 50±5 ms, compared with 1.5 s for pBASEX51, 4.86 s for POP53and 174 s for the iterative procedure52. For a full-sized 1040 × 1054 pixel image, the inversion time was still only around 600 ms, well below the image acquisition time. Additional efficiency was gained by separating the image acquisition and analysis steps. Thus, while one image was being acquired, the previous image was being inverted. As the exposure time is almost always longer than the image processing time, the overall time for the experiment was not affected by the addition of the inversion step into the control loop. Figure 7: Comparison of raw 2D and processed 3D images. The raw ( a ) and rapidly inverted ( b ) images for CD 3 + ions. The inversion was accomplished with the ‘onion-peeling’ or ‘back-projection’ method described in this section. The purple and white boxed regions in ( b ) illustrate how different processes could be isolated from the CD 3 + images and the corresponding yields used to define a control objective. On a 661 × 661 pixel test image, our algorithm could produce an inverted image in 50±5 ms, compared with 1.5 s for pBASEX [51] , 4.86 s for POP [53] and 174 s for the iterative procedure [52] . For a full-sized 1040 × 1054 pixel image, the inversion time was still only around 600 ms, well below the image acquisition time. Additional efficiency was gained by separating the image acquisition and analysis steps. Thus, while one image was being acquired, the previous image was being inverted. As the exposure time is almost always longer than the image processing time, the overall time for the experiment was not affected by the addition of the inversion step into the control loop. Full size image Mathematically, given the cylindrical symmetry conveniently provided by the laser polarization axis, accomplishing the image inversion requires performing an inverse Abel transformation [22] , [45] , [46] , [47] . A number of numerical methods for solving this problem exist, but not all of them are useful for this rapid online inversion owing to the additional constraints of the adaptive control loop. First, as a typical experiment contains a few thousand trial pulses, the inversion cannot take much longer than the image acquisition time. Ideally, the inversion time will be much shorter. Second, as the image features are not known ahead of time, methods that require manual selection of initial parameters (such as an appropriate basis set) are difficult to implement. Finally, the inversion process should avoid introducing noise that compromises the feedback. Inversion selection and speed tests With these constraints in mind, it is worth reviewing a few options. Fourier–Hankel-based methods [48] , [49] can be quite rapid but can often result in increased noise, especially near the centre of the image where the Bessel function oscillates rapidly [22] . Several methods, such as BASEX [50] and pBASEX [51] , take advantage of the fact that some functions have known inverse Abel transformations. These methods have several advantages, including a relocation of the centerline noise common to the Abel methods to the centre point of the image, relatively rapid computation and smooth final images. The main drawback for our application is that they require the selection of a basis set before the experiment. An alternative approach, which converges to the measured 2D projection by making iterative guesses about the 3D distribution, was developed by Vrakking [52] but is significantly slower. In recent years, several hybrid methods have appeared, including a polar onion peeling (POP) [53] approach that uses a basis set technique similar to BASEX, and an approach that combines BASEX-like features with the iterative approach [54] . These also had undesirable features for our online processing application, primarily the need to set initial values of some kind. In addition, the POP algorithm produced negative values in our tests, which significantly complicates the determination of a yield-based fitness value. For these reasons, we selected the well-known ‘onion-peeling’ or ‘back-projection’ method [22] , [30] . Although this technique does result in some centerline noise, it is typically less significant than with the Fourier–Hankel methods, and the noise can be reduced to minimal levels. Importantly, there are no initial parameters to be specified, other than the centre and size of the image. Our implementation was derived from the algorithm described by Bordas and co-workers [30] , and the interested reader is directed to their excellent development of the mathematical formalism. Careful optimization of our implementation of this method reduced the computation time for our 661 × 661 pixel test image to 50 ms, shorter than any other method we tested. The overall image processing time is typically less than the duration of the image acquisition, and therefore the overall time of the experiment is not affected. Pulse parameterization In most of these experiments the spectral phase was controlled via sixteen ‘genes’ spread over the pulse bandwidth. The spectral phases between adjacent gene values are calculated by linear interpolation. The time-domain parameterization method allows the shaped pulse to be built out of a series of n Gaussian-shaped pulses [18] . In an example where the full pulse is composed of three component pulses, eight genes are needed: three amplitudes ( a 1 , a 2 and a 3 ), three pulse durations ( w 1 , w 2 and w 3 ) and two time delays ( t 12 and t 13 ). To obtain the phase mask needed to produce the desired laser intensity as a function of time while only controlling the spectral phase delay, we used the algorithm developed by Hacker and co-workers [55] . This algorithm rapidly estimates the needed phase mask using a process that iteratively employs a FFT-based approach. FTL fitness determination The degree of control is reported with respect to the value of the fitness function obtained with a FTL pulse. Experimentally, between each generation an FTL pulse is tested under the same conditions as the trial pulse. These results are averaged over the entire experiment to produce the baseline value that serves as a comparison for the shaped pulses. The fluctuations in the FTL fitness value obtained during each experiment define σ for that experiment. Selection of regions of interest Generally, images of various fragmentation channels are obtained with FTL pulses and these results are used to make an initial selection of a feature for optimization. In the acetylene example, previous results [31] , [32] were also used to inform our selection. Features will often shift in energy or angular distribution as different laser pulse shapes are applied, so selecting too restrictive of a region for use in calculating the fitness function can lead to difficulties with the search. In fact, too restrictive of a gate on the CH 2 + image shown in Fig. 2a,b did lead to spurious results by excluding lower KER ions from the fitness calculation. In this particular case, however, extending the gate lower in KER than shown in Fig. 2a,b did not affect the results. Ethylene calculations As described more fully in ref. 39 , the angular-dependent ionization probabilities for ethylene are calculated based on the electronic structure theory. To describe the interaction between the laser pulse and the molecule, the polarization is fixed and the molecule is rotated around that plane as well as out of the plane, that is, around the C=C bond direction. For each position, the electronic wave function is calculated in the presence of the electric field and the tunnelling probability is deduced for the various orbitals. Ionization from more than a single molecular orbital is treated using a linear combination of the selected orbitals. Acetylene calculations The 2D PES of C 2 H 2 2+ ( ) was calculated on the CASSCF [8] , [10] level with a 6-311++G** basis set using the programme package MOLPRO [56] . The scan was carried out under relaxation of the remaining coordinates. The acetylene trajectories were calculated on the same level of theory and utilized an adapted version of the NewtonX program package [57] for the on-the-fly interface to MOLPRO. Trajectories were calculated for the and states. They show similar topography and can be reached in the ionization process. To include the effect of the remaining laser field after ionization, we first checked for possible interaction pathways via electronic excited states that could be used for laser-based control. No electronic excited states can be reached with the laser frequency (or are symmetry forbidden) for both the singlet and the triplet states of the dication. The possibility of two photon transitions was also considered following the approach of ref. 58 , but could be excluded. For the FTL laser pulse we assumed a Wigner distribution in the Franck–Condon region of the molecule with excess energy from the laser distributed in the vibrational modes [59] , [60] . Here, we assumed that the first half of the laser pulse is needed for ionization. For the optimal laser pulse, we took the experimental field and assumed that ionization occurred around the maximum of the first sub-pulse. After ionization the trajectories started again from individual points of a Wigner distribution in the Franck–Condon region. The remaining laser pulse was then added to the one-electron Hamiltonian at the distinct time steps and was included in the on-the-fly dynamics. How to cite this article: Wells, E. et al. Adaptive strong-field control of chemical dynamics guided by three-dimensional momentum imaging. Nat. Comm. 4:2895 doi: 10.1038/ncomms3895 (2013).